Asymmetric trapping of zwitterionic intermediates by sulphur ylides in a palladium-catalysed decarboxylation-cycloaddition sequence Through nearly 50 years of development, sulphur ylides have been established as versatile and powerful reagents for the construction of carbocycles and heterocycles. Despite advances, two important and yet elusive bottlenecks continue to inhibit the advancement of this chemistry: a limited number of reagents with polar groups to react with sulphur ylides, and the wide utilization of chiral auxiliaries or substrates to achieve asymmetric cycloaddition processes in the majority of known reports. Herein, we apply an asymmetric palladium catalysis strategy to the chemistry of sulphur ylides to address these two fundamental problems. We thus achieve an unprecedented decarboxylation-cycloaddition sequence of cyclic allylic esters with sulphur ylides through the enantioselective trapping of Pd-stabilized zwitterionic intermediates by the ylides. As a result, a series of biologically and synthetically important 3-vinyl indolines are rapidly assembled with a high reaction efficiency and stereoselectivity. A sulphur ylide is a neutral dipolar molecule containing a carbanion and an adjacent sulphonium cation [1] . Because of their unique nucleophilic and then electrophilic reactivity, sulphur ylides are usually used as a versatile methylene synthon not only in synthetic laboratories [2] but also in many bacteria [3] , [4] , [5] . For example, in the well-known Johnson–Corey–Chaykovsky reaction [6] , which was first discovered in the 1960s (refs 7 , 8 ), sulphur ylides can react with polar substrates (for example, aldehydes, ketones, imines and electron-deficient alkenes) to produce a wide range of significant small-ring molecules such as epoxides, aziridines and cyclopropanes. More importantly, their synthetic potential has been well demonstrated in the synthesis of numerous bioactive natural products and pharmaceuticals [6] , [9] , [10] . In the past decade, the cycloaddition chemistry of sulphur ylides has evolved dramatically beyond three-membered rings, largely as a consequence of the valuable contributions made by Aggarwal and co-workers [11] , [12] , [13] , [14] , [15] , [16] , [17] , [18] , [19] , [20] , [21] , [22] , among others. For instance, in 2006, Aggarwal’s group developed an elegant epoxy-annulation sequence reaction of vinyl sulphonium salts, which are important precursor of sulphur ylides, to rapidly convert aminoaldehydes, ketones and imines into epoxide-fused heterocycles ( Fig. 1a ) [13] . Significantly, a nine-step synthesis of (−)-balanol, an important protein kinase C inhibitor, was achieved starting from a chiral tert -butyl sulphinimine, with this methodology as a key step. Another impressive example was published by Tang’s laboratory, who, in 2008, reported a highly efficient synthesis of cyclohexadiene epoxides via a tandem ylide Michael addition/epoxidation reaction of α,β-unsaturated ketones with crotonate-derived sulphonium salts ( Fig. 1b ) [14] . They achieved high enantioselectivities and diastereoselectivities by employing camphor-derived chiral sulphonium salts. In the same year, our own group developed a cascade reaction involving acyl-stabilized sulphur ylides and nitroolefins—specifically, a [4+1] cycloaddition/rearrangement cascade ( Fig. 1c ) [15] , [16] . Notably, chiral H-bonding catalysis was successfully applied to this transformation, affording enantio-enriched oxazolidin-2-one products in good efficiency and selectivity. Furthermore, the natural isolates valinoctin A and (−)- epi -cytoxazone with important biological activities were obtained through this cascade reaction. Despite impressive advances, the chemistry of sulphur ylides has still not achieved its full potential. Until very recently, π-Lewis-acid-gold complex-assisted cycloadditions of sulphur ylides with electron-neutral alkynes [17] , [18] and alkenes [19] have been sporadically reported. However, limited success has been achieved using catalytic asymmetric technologies to achieve asymmetric cycloadditions of sulphur ylides [16] , [20] , [21] , [22] . In general, stoichiometric amounts of chiral auxiliaries or starting materials are required in the majority of reports to ensure good reaction efficiency and stereo-control. Therefore, the search for efficient asymmetric catalytic technologies and novel organic transformations of sulphur ylides, with the goal of increasing the diversity of the substrates and products, is still highly desirable. 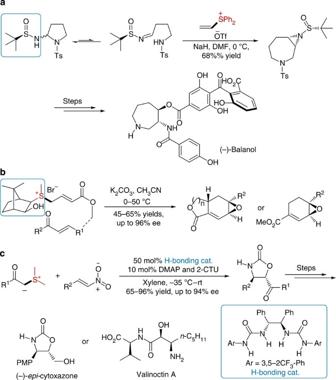Figure 1: Selected examples. (a) Aggarwal’s work with vinyl sulphonium salts. (b) Tang’s work with crotonate-derived sulphonium salts. (c) Our work with acyl-stabilized sulphur ylides. DMAP:N,N-dimethylpyridin-4-amine; 2-CTU: 1-(2-chlorophenyl)thiourea. Figure 1: Selected examples. ( a ) Aggarwal’s work with vinyl sulphonium salts. ( b ) Tang’s work with crotonate-derived sulphonium salts. ( c ) Our work with acyl-stabilized sulphur ylides. DMAP: N , N -dimethylpyridin-4-amine; 2-CTU: 1-(2-chlorophenyl)thiourea. Full size image Palladium-catalysed decarboxylation-cycloaddition (DC) reactions of cyclic allylic esters ( Fig. 2a , A ) have grown at a rapid pace in recent years [23] , [24] , [25] , [26] . The key to these successes is the in situ generation of the common Pd-stabilized zwitterionic intermediates B . From the perspective of reaction mechanisms, the nucleophilic part ( X − : nitrogen or α-carbonyl anion) of these intermediates first reacts with electrophilic reagents such as electron-deficient alkenes, 1,3-dipoles and isocyanates and simultaneously affords new zwitterionic intermediates C . Subsequently, intramolecular allylations of the anion part ( N − ) by the electrophilic π-allylpalladium component deliver final cyclization products D . Through this nucleophilic addition (NuD) followed by electrophilic addition (ElD) process, a wide range of five-, six- and seven-membered ring compounds were efficiently constructed. In contrast, we wonder whether the apparent reversal of the ambident reactivity of these zwitterionic species could be used to further exploit novel cyclization reactions of cyclic allylic esters with nucleophilic reagents. 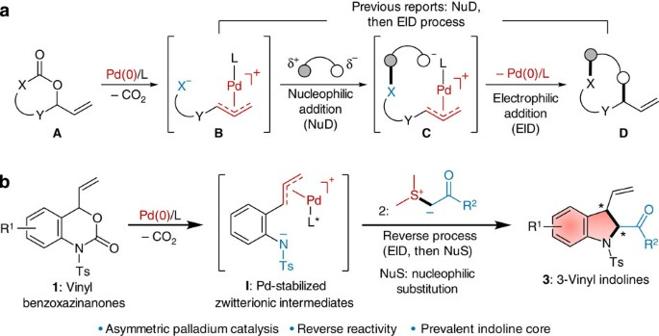Figure 2: Reaction design. (a) Previous reports: trapping of Pd-stabilized zwitterionic intermediates by electrophilic reagents for the decarboxylation-cyclization sequence. (b) This work: trapping of Pd-stabilized aza-o-xylylenes by nucleophilic sulphur ylides. Figure 2: Reaction design. ( a ) Previous reports: trapping of Pd-stabilized zwitterionic intermediates by electrophilic reagents for the decarboxylation-cyclization sequence. ( b ) This work: trapping of Pd-stabilized aza- o -xylylenes by nucleophilic sulphur ylides. Full size image In the past several years, we are interested in carbo- and heterocycle synthesis by using acyl-stabilized sulphur ylides [12] , [15] , [16] , [27] , [28] , [29] . We herein describe an unprecedented Pd-catalysed DC reactions of vinyl benzoxazinanones by using sulphur ylides to highly enantioselectively trap Pd-stabilized zwitterionic intermediates I ( Fig. 2b ). Notably, trapping of these intermediates with electrophilic components for cycloaddition was hitherto unknown and remains a challenging goal in this field of Pd-catalysed DC reactions because, as Tunge concluded, “…palladium-polarized aza-ortho-xylylenes (D) (note: intermediate I here) prefer to react with electron deficient olefins…” [30] . More significantly, via this approach, an important indoline core that is ubiquitous in many biologically active natural and synthetic chemicals could be conveniently constructed in a highly enantioselective and diastereoselective manner [31] , [32] , [33] . The method described here is a complement to previous efficient protocols including kinetic resolutions of racemic indolines [34] , catalytic asymmetric hydrogenation of indoles [35] and de nevo construction of chiral indolines via formal [3+2] cycoloaddions of anilines and olefins [36] . Optimization of reaction conditions The feasibility of this planned Pd-catalysed DC reaction was examined using vinyl benzoxazinanone 1a (1.0 equiv.) and sulphur ylide 2a (2.0 equiv.) in dichloromethane at room temperature. Notably, no reaction occurred in the absence of the Pd catalyst as shown in Fig. 3 . The addition of a catalytic amount of [Pd(PPh 3 ) 4 ] (10 mol%) promoted the synthesis of the desired indoline product in good isolated yield and with high selectivity (77% yield, >95:5 diastereomer ratio (d.r.)). Encouraged by this initial result, we turned our attention to the development of Pd-catalysed asymmetric DC reactions. Initially, Trost’s ligands ( Table 1 , L1 and L2 ) [37] together with Pd 2 (dba) 3 ·CHCl 3 (5 mol%, dba: dibenzylideneacetone) were tested for the model reaction. These reaction conditions resulted in detectable enantioselectivities, moderate yields and complete diastereo-control ( Table 1 , entries 1 and 2: 55% yield, >95:5 d.r., 20% enantiomeric excess (e.e.) and 64% yield, >95:5 d.r., 8% e.e.). A series of chiral ligands ( L3 – L8 ) were then evaluated for this asymmetric DC reaction. As summarized in Table 1 , BINOL-derived chiral phosphoramidites ( L4–L6 , BINOL: 1,1′-binaphthalene-2,2′-diol) [38] exhibited better enantiocontrol capacity ( Table 1 , entries 4–6) than the others ( Table 1 , entries 1–2 and 7–8). The palladium complex with You’s chiral ligand L6 (ref. 39 ) promoted this reaction with remarkably high efficiency and enantioselectivity ( Table 1 , entry 6: 99% yield, >95:5 d.r. and 83% e.e.). Other palladium sources were also screened, and Pd 2 (dba) 3 and Pd(acac) 2 (acac: acetylacetonate) gave similar results in terms of both efficiency and selectivity. Afterwards, further efforts were made to improve the enantioselectivity. A significant solvent effect on enantioselectivity was observed, and chloroform was the solvent of choice ( Table 1 , entry 12: 99% yield, >95:5 d.r., 89% e.e.). In addition, the enantiocontrol could be further improved when the reaction was conducted at −40 °C, although a prolonged reaction time was needed. The reaction efficiency and selectivity were retained when the amount of sulphur ylide was reduced to 1.5 equiv. ( Table 1 , entry 17: 95% yield, >95:5 d.r., 94% e.e.). 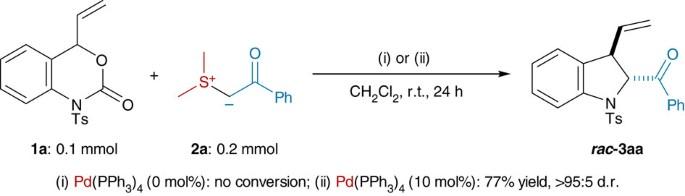Figure 3: Initial results. (i) No reaction occurred in the absence of the Pd catalyst. (ii) The desired product generated smoothly in the presence of Pd(PPh3)4. Figure 3: Initial results. (i) No reaction occurred in the absence of the Pd catalyst. (ii) The desired product generated smoothly in the presence of Pd(PPh 3 ) 4 . Full size image Table 1 Condition optimization of Pd-catalysed asymmetric DC reactions of vinyl benzoxazinanone 1a with sulphur ylide 2a . Full size table Substrate scope With the optimum reaction conditions established, a variety of substrate combinations were evaluated to define the scope of Pd-catalysed asymmetric DC reactions. As highlighted in Table 2 , a number of substituted benzoyl-stabilized sulphur ylides were determined to be suitable for this reaction. Variations of the electronic and steric properties of the substituents on the benzene ring had little effect on the reaction efficiency or stereoselectivity ( Table 2 , entries 1–6:≥90% yield, >95:5 d.r. and up to 96% e.e. ); the exception was the meta -Br-substituent ( Table 2 , entry 7: 75% yield, >95:5 d.r. and 96% e.e. ), which resulted in a slightly lower yield. Heteroaryl-substituted acyl sulphur ylides (that is, 2-furanyl and 2-thiophenyl) were also useful reactants, providing the corresponding indoline products in high yields and with high stereoselectivities ( Table 2 , entries 8 and 9: 79% yield, >95:5 d.r. and 91% e.e. ; 86% yield, >95:5 d.r. and 99% e.e.). Moreover, the scope of sulphur ylides can be significantly extended to alkoxyl-, alkenyl- and alkyl-acyl-substituted ones ( Table 2 , entries 10–12: 81–91% yields, >95:5 d.r. and up to 93% e.e.). Table 2 Survey of the vinyl benzoxazinanone and sulphur ylide scope in the Pd-catalysed asymmetric DC reactions. Full size table From the perspective of product diversity, a wide range of vinyl benzoxazinanones were examined for the cycloaddition reaction of representative benzoyl- ( 2a ) and ester-stabilized sulphur ylides ( 2j ). As shown in Table 2 , benzoxazinanone substrates with electron-rich and electron-deficient substitutes were compatible, being successfully converted into various indoline products with good results ( Table 2 , entries 13–15 and 19–21: 81–98% yields, >95:5 d.r. and up to 98% e.e.). Furthermore, this Pd-catalysed asymmetric DC reaction also tolerated variation of the position of the substituent on the benzene ring of vinyl benzoxazinanones, producing the corresponding indoline products in satisfactory isolated yields and stereoselectivities ( Table 2 , entries 16–18 and 22–24: 62–96% yields, >95:5 d.r. and up to 95% e.e.). Notably, the incorporation of diverse halogen functional groups into the desired indoline products holds potential for further synthetic modifications through organometallic technologies [40] , [41] . Synthetic versatility of reaction methodology We then conducted a gram-scale reaction using the present chiral palladium catalysis system ( Fig. 4a ). No obvious erosive effect on reaction efficiency or selectivity (91% yield, >95:5 d.r. and 93% e.e.) was observed. Moreover, the conventional synthetic operation can further enrich the diversity of the vinyl segment through the use of our previous cross-metathesis reaction conditions [42] . For example, chiral indoline 3aa was transformed to methyl and tert -butoxyl ester-substituted products ( Fig. 4b,c ) in good yields and with high optical purities in the presence of a catalytic amount of Ru metathesis catalyst and Lewis acid. 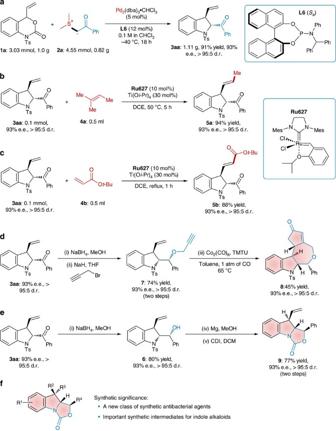Figure 4: Evaluating the potential of this strategy to address synthetically relevant problems. (a) Gram-scale reaction. (b,c) Application of the cross-metathesis (CM) reaction to introduce other substituents at the end of a terminal alkene. (d,e) Derivatization of chiral indoline product3a. (f) Synthetic significance of the oxazolo[3,4-a]indol-3-one core. Reagents and conditions: (i) NaBH4(4 equiv.), MeOH, 0 °C, 30 min, then room temperature (r.t.), 2 h; (ii) NaH (1.5 equiv.), propargyl bromide (1.3 equiv.), THF, r.t., 5 h; (iii) Co2(CO)8(0.3 equiv.), TMTU (1.2 equiv.), CO (1 atm), toluene, 65 °C, 4 h; (iv) Mg (powder, 10 equiv.), MeOH, N2, 12 h; (V) CDI (1.1 equiv.), DCM, r.t., 12 h. TMTU: tetramethyl thiourea; CDI: di(1H-imidazol-1-yl)methanone. Figure 4: Evaluating the potential of this strategy to address synthetically relevant problems. ( a ) Gram-scale reaction. ( b , c ) Application of the cross-metathesis (CM) reaction to introduce other substituents at the end of a terminal alkene. ( d , e ) Derivatization of chiral indoline product 3a . ( f ) Synthetic significance of the oxazolo[3,4-a]indol-3-one core. Reagents and conditions: (i) NaBH 4 (4 equiv. ), MeOH, 0 °C, 30 min, then room temperature (r.t.), 2 h; (ii) NaH (1.5 equiv. ), propargyl bromide (1.3 equiv. ), THF, r.t., 5 h; (iii) Co 2 (CO) 8 (0.3 equiv. ), TMTU (1.2 equiv. ), CO (1 atm), toluene, 65 °C, 4 h; (iv) Mg (powder, 10 equiv. ), MeOH, N 2 , 12 h; (V) CDI (1.1 equiv. ), DCM, r.t., 12 h. TMTU: tetramethyl thiourea; CDI: di(1 H -imidazol-1-yl)methanone. Full size image To further demonstrate the synthetic potential of this approach, the indoline product 3aa was subjected to other transformations ( Fig. 4d–f ). For example, reduction with sodium borohydride followed by propargylation gave 7 in high yield and selectivity (74% yield, >95:5 d.r. and 93% e.e. for two steps). Then, a Pauson–Khand reaction with a cobalt catalyst under a CO atmosphere [43] afforded the complex molecule 8 (45% isolated yield, 93% e.e. and >95:5 d.r.). This structure features a fused carbo-/heterocyclic architecture as well as a challenging seven-membered ring. Moreover, after chiral indoline 3aa was reduced, a two-step operation including the deprotection of the tosyl group with magnesium powder and treatment with CDI provided the desired product 9 with an oxazolo[3,4- a ]indol-3-one core (77% isolated yield, 93% e.e. and >95:5 d.r. in two steps). Significantly, this family of oxazolo[3,4- a ]indol-3-ones exhibits significant synthetic value ( Fig. 4f ) [44] , [45] , not only as a new class of potent antibacterial agents but also as important intermediates in the synthesis of natural indoline alkaloids. The optical purities of the compounds were not affected in these synthetic transformations, and new stereocentres were generated in good diastereoselectivities, which we established unambiguously using Nuclear Overhauser Enhancement Spectroscopy spectra. A possible mechanism for this Pd-catalysed asymmetric DC reaction is shown in Fig. 5a . Initially, Pd-polarized aza- o -xylylene I was obtained from substrate 1a through a decarboxylation reaction promoted by the chiral Pd 0 catalyst (generated in situ from a Pd 0 source and chiral phosphoramidite L6 ). Next, this species reacted with sulphur ylide 1a to form Pd complex II through electronic interaction. A new C–C bond was formed irreversibly via an intramolecular asymmetric allylation reaction, and the new intermediate III was generated in good regioselectivity and stereoselectivity. The subsequent decomposition of this species resulted in the regeneration of the chiral Pd 0 catalyst and the simultaneous formation of the zwitterionic species IV . Finally, the desired chiral indoline product 3aa was achieved through bond rotation and N -alkylation. The electrostatic interaction between the positive sulphonium ion and negative sulphamide anion was believed to play a pivotal role in the complete branched regioselectivity and good enantioselectivity (see the stereochemistry analysis in Fig. 5c,d ). Although it has been demonstrated in previous work [46] , this weak interaction was further confirmed by the control experiments. For example, when an electrolyte was introduced into the standard condition, the Pd-catalysed asymmetric DC reaction was completely inhibited (LiBr) or its conversion and enantioselectivity were severely affected (Bu 4 N + Br − ), perhaps because the electrostatic interaction in the key intermediate II ( Fig. 5b ) might be subjected to interference by the additional electrolyte. 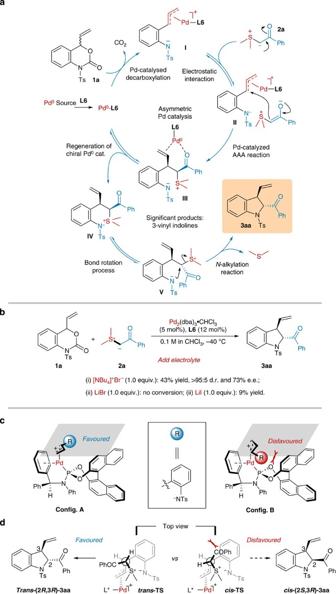Figure 5: Mechanism and stereochemistry analysis. (a) Our proposed reaction mechanism. (b) Electrolyte effects. (c) Proposed configurations of chiral Pd-polarized aza-o-xylylene (I). (d) Proposed transition states (Newman projection of the top view). Figure 5: Mechanism and stereochemistry analysis. ( a ) Our proposed reaction mechanism. ( b ) Electrolyte effects. ( c ) Proposed configurations of chiral Pd-polarized aza- o -xylylene ( I ). ( d ) Proposed transition states (Newman projection of the top view). Full size image The combination of Pd and BINOL-derived chiral phosphoramidites has been developed into a privileged catalyst in asymmetric organic transformations [39] over the past 20 years. Significantly, many reactive Pd-allyl phosphoramidite complexes have been isolated, and their configurations have been established through X-ray diffraction (see Supplementary Fig. 40 ) and two-dimensional (2D) NMR technologies [47] , [48] . On the basis of these advances, we proposed a favourable configuration ( Fig. 5c , Config. A ) for key intermediate I , as depicted in Fig. 5c ; this configuration avoids the steric repulsion between the tosyl aniline component and the binaphthyl skeleton ( Fig. 5c , Config. B ). Because the bottom of this intermediate ( Config. A ) was blocked, the attack of the sulphur ylide 1a was assumed to be more favourable. It is well known that both dipole–dipole interactions and the steric hindrance of torsional rotations are critical to control the high E -selectivity and diastereoselectivity in the epoxide formation from sulphur ylides and the Wittig reaction of stabilized phosphonium ylides [46] , [49] . Accordingly, two Newman projections of possible transition states can be considered on the basis of electrostatic interactions ( Fig. 5d , top view). In addition, we speculated that the indoline product trans-( 2 R, 3 R)- 3aa and its epi -isomer cis-( 2 R, 3 R)- 3aa could result from trans -TS and cis -TS , respectively, followed by bond rotation and N -alkylation processes. However, the former was believed to be more favourable than the latter because of its lower steric hindrance. This explanation of the stereochemistry is somewhat supported by the absolute configuration of cycloadduct 3aa , which was confirmed by XRD analysis. It is worthy to note that other possibilities for the high diastereoselectivity cannot be ruled out at the current stage. For example, reversible proton transfer of intermediate IV / V dynamically favours the diastereomer to undergo fast ring-closing step; the slow keto–enol tautomerism under basic condition thermodynamically favours trans -configuration product, which has been supported by the D 2 O experiment (see Supplementary Fig. 41 ). In conclusion, we have achieved an enantioselective trapping of palladium-stabilized zwitterionic intermediates with nucleophilic dipole sulphur ylides for the first time. An unprecedented Pd-catalysed asymmetric decarboxylation-cyclization sequence of sulphur ylide with vinyl benzoxazinanones was achieved, providing a wide range of significant 3-vinyl indoline products in good reaction efficiencies (62–99% yields) and stereoselectivities (up to >95:5 d.r. and 99% e.e.). Notably, via the asymmetric palladium catalysis technology described here, the cycloaddition chemistry of the sulphur ylides was significantly extended to non-polar reagents, specifically, cyclic allylic esters. Moreover, the corresponding asymmetric cycloaddition process also occurred in the presence of a catalytic amount of chiral ligand. Therefore, we believe this work will open new avenues for reaction design and carbocycle/heterocycle synthesis based on these versatile and powerful sulphur ylides. Materials Unless otherwise noted, materials were purchased from commercial suppliers and used without further purification. All the solvents were treated according to standard methods. Flash column chromatography was performed using 200–300 mesh silica gel. All air- and moisture-sensitive reactions were performed under an atmosphere of N 2 in fire-dried glassware. The manipulations for Pd-catalysed reactions were carried out with standard Schlenk techniques under Ar. See Supplementary Methods for details. General spectroscopic methods 1 H NMR spectra were recorded on 400 or 600 MHz spectrophotometers. 13 C NMR spectra were recorded on 100 or 150 MHz with complete proton-decoupling spectrophotometers (CDCl 3 : 77.0 p.p.m.). High resolution mass spectrometry (HRMS) was recorded on Agilent technologies 6224 time of flight (TOF) liquid chromatography-mass spectrometry (LC/MS) instrument or Bruker ultrafleXtreme matrix-assisted laser desorption/ionization–TOF (MALDI-TOF)/TOF mass spectrometer. e.e. values were determined by chiral HPLC with chiral columns (chiralpak AS-H column, chiralpak AD-H column, chiralpak OJ-H column, chiralpak IC-H column or chiralcel OD-H column) with hexane and i -PrOH as solvents. Optical rotations were measured with a polarimeter. 1 H NMR, 13 C NMR and HPLC spectra are supplied for all compounds: see Supplementary Figs 1–39 and Supplementary Table 1 . See Supplementary Methods for the characterization data of all compounds related. General procedure for Pd-catalysed asymmetric DC reactions In a flame-dried Schlenk tube under N 2 , Pd 2 (dba) 3 ·CHCl 3 (0.01 mmol, 10.35 mg) and phosphoramidites ligand L6 (0.024 mmol, 12.6 mg) were mixed in dry chloroform and stirred at room temperature for 20 min. The mixture was then cooled to −40 °C, and vinyl benzoxazinanone 1a (0.2 mmol, 66 mg) and sulphur ylide 2a (0.3 mmol, 54 mg) were successively introduced. The resulting dark-green solution was stirred at this temperature until the reaction was completed (as indicated by thin-layer chromatography). After the solvent was evaporated under reduced pressure, the crude product was purified via flash chromatography (SiO 2 , 12:1 petroleum ether:ethyl acetate) to give chiral 3-vinyl indoline 3aa as a white solid. d.r. is >95:5, as determined by 1 H NMR of the reaction mixture. e.e. is 94%, as determined by HPLC (Daicel Chirapak AD, hexane/isopropanol=70/30, flow rate 1.0 ml min −1 , T=25 °C, 254 nm): t R =13.175 min (major), t R =21.88 min (minor), (c=1.0, CHCl 3 ). How to cite this article: Li, T.-R. et al . Asymmetric trapping of zwitterionic intermediates by sulphur ylides in a palladium-catalysed decarboxylation-cycloaddition sequence. Nat. Commun. 5:5500 doi: 10.1038/ncomms6500 (2014). Accession codes: The X-ray crystallographic coordinates for structures reported in this Article have been deposited at the Cambridge Crystallographic Data Centre (CCDC), under deposition numbers CCDC 1009688. These data can be obtained free of charge from The Cambridge Crystallographic Data Centre via http://www.ccdc.cam.ac.uk/data_request/cif .